Mitochondrial reactive oxygen species regulate the strength of inhibitory GABA-mediated synaptic transmission Neuronal communication imposes a heavy metabolic burden in maintaining ionic gradients essential for action potential firing and synaptic signalling. Although cellular metabolism is known to regulate excitatory neurotransmission, it is still unclear whether the brain’s energy supply affects inhibitory signalling. Here we show that mitochondrial-derived reactive oxygen species (mROS) regulate the strength of postsynaptic GABA A receptors at inhibitory synapses of cerebellar stellate cells. Inhibition is strengthened through a mechanism that selectively recruits α3-containing GABA A receptors into synapses with no discernible effect on resident α1-containing receptors. Since mROS promotes the emergence of postsynaptic events with unique kinetic properties, we conclude that newly recruited α3-containing GABA A receptors are activated by neurotransmitter released onto discrete postsynaptic sites. Although traditionally associated with oxidative stress in neurodegenerative disease, our data identify mROS as a putative homeostatic signalling molecule coupling cellular metabolism to the strength of inhibitory transmission. Although the mammalian brain represents a small fraction of the total body mass, its energy requirements are substantial. Most neural energy is expended on sustaining excitatory signalling within the central nervous system [1] with action potential firing and glutamatergic transmission proposed to contribute as much as 80% of total expenditure [2] . Such high requirements, combined with limited energy reserves, place limits on the size of the evolving brain [3] obliging neuronal circuits to develop metabolically-efficient wiring [4] and signalling [5] , [6] strategies. How energy consumption is then distributed among different cell types is still unclear, although most work has focused on excitatory principal neurons and astrocytes [7] , [8] , [9] . While the bioenergetics of inhibitory GABAergic interneurons has received less attention [10] , emerging data suggest a similar high demand on cellular metabolism. Inhibitory stellate and basket cells of the cerebellum, for example, are computed to use almost half their energy on postsynaptic receptor signalling [11] placing them on par with the energy demands of principal neurons such as Purkinje cells. In keeping with this, GABAergic transmission at cerebellar stellate cells is particularly robust [12] , [13] implying that a significant proportion of energy is expended on reversing ion-gradients generated by synaptic activity. In fact, stellate cells are a particularly attractive model cell in which to study coupling of cellular metabolism with inhibitory transmission for two reasons. First, inhibitory transmission at stellate cells is relatively stable over time in terms of synaptic event amplitude and frequency making it ideal for quantitative analyses [13] , [14] . Second, prior work has established that stellate cell inhibitory synapses contain GABA A receptors of known composition which would be helpful in dissecting the molecular nature of any regulatory mechanism. Inhibitory stellate cell synapses of the young adult cerebellum contain GABA A receptors composed of α1, β2 and γ2 subunits [15] , [16] . α2- and/or α3-containing GABA A receptors may also play a minor role but their contribution is thought to diminish during development [17] , [18] . Here we have used the stellate cell inhibitory synapse to examine whether cellular metabolism regulates GABAergic signalling. Electrophysiological recordings demonstrate that GABAergic synapse strengthening occurs through a novel mechanism where mitochondrial-derived reactive oxygen species (mROS) recruit α3-containing GABA A receptors. Interestingly, mROS do not strengthen established synapses that contain α1-receptors. Taken together, our work highlights an unexpected role for mROS in signalling the metabolic state of the cell to the inhibitory synapse. Antimycin-A increases GABAergic synaptic event frequency To determine whether inhibitory transmission is coupled to the metabolic state of the postsynaptic cell, we performed voltage-clamp recordings of miniature inhibitory postsynaptic currents (mIPSCs) that are mediated by GABA A receptors in cerebellar stellate cells. In agreement with other studies, our data revealed that event frequency and amplitude changed little during a typical 25–30 min recording ( Fig. 1 ). For a more quantitative analysis, event frequency and amplitude were compared in each recording from synaptic events detected during the first (0–5) and last (20–25) 5 min ( Fig. 1a ) after seal breakthrough. Fits of the amplitude distributions from stellate cells ( n =6) revealed that most tetrodotoxin (TTX)-insensitive GABAergic events were best fitted by 3 to 4 Gaussian components. For example, detected events from the first 5 min of the recordings gave peak values of −42 pA (13.7%), −75 pA (61.7%) and −139 pA (24.6%) ( Fig. 1b , left). Similar fits were obtained with data obtained from the last 5 min of the recording after seal breakthrough ( Fig. 1b , right), highlighting that inhibitory transmission is stable under these recording conditions. 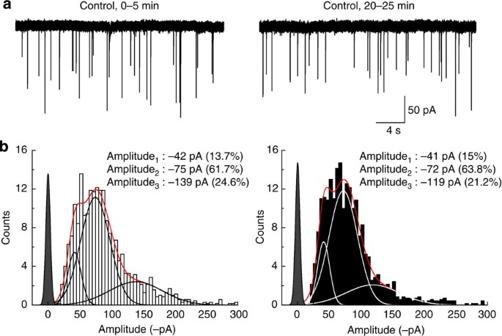Figure 1: Inhibitory transmission onto cerebellar stellate cells is stable. (a) mIPSCs recorded from the same stellate cell (cell no. 120202p2) at two time periods showing that event amplitude and frequency were similar throughout. (b) Amplitude distributions of inhibitory events from stellate cell recordings (n=6) comparing early (i.e., 0–5 min) and later (i.e., 20–25 min) events. Averaged data has been fit with the sum of three Gaussian functions (red line) with individual Gaussians shown in either black (left panel) or white (right panel). In this figure and other figures, closed point distribution (filled) has been scaled to the fitted peak of the lowest event amplitude and represents the average noise observed during the recordings. Figure 1: Inhibitory transmission onto cerebellar stellate cells is stable. ( a ) mIPSCs recorded from the same stellate cell (cell no. 120202p2) at two time periods showing that event amplitude and frequency were similar throughout. ( b ) Amplitude distributions of inhibitory events from stellate cell recordings ( n =6) comparing early (i.e., 0–5 min) and later (i.e., 20–25 min) events. Averaged data has been fit with the sum of three Gaussian functions (red line) with individual Gaussians shown in either black (left panel) or white (right panel). In this figure and other figures, closed point distribution (filled) has been scaled to the fitted peak of the lowest event amplitude and represents the average noise observed during the recordings. Full size image To directly test the impact of cellular metabolism on inhibitory transmission, we performed identical experiments but included antimycin-A in the patch pipette solution to disrupt mitochondrial function. Prior biochemical studies have established the selective effect of antimycin-A on the mitochondria, where it concurrently blocks ATP production and generates the free radical superoxide [19] . This pharmacological effect is achieved by inhibiting cytochrome c reductase, which disrupts the proton gradient needed by ATP synthase to make ATP [20] . Electrons made available by antimycin-A permit the formation of superoxide. Inclusion of 2 μM antimycin-A in the patch pipette had an almost immediate effect on synaptic events mediated by GABA A receptors ( Fig. 2 ). Unlike the control condition, the frequency of mIPSCs increased significantly over the duration of the recording ( Fig. 2a ). During the first 5 min, the total event frequency (mean±s.e.m.) was 1.10±0.07 Hz which increased to 1.78±0.08 Hz after 20–25 min ( n =5; P =7.1 × 10 −9 , paired, two-tailed Student’s t -test). Gaussian fits of the amplitude distributions revealed that the increase in frequency was almost exclusively limited to synaptic events of smaller amplitudes (i.e.,<−100 pA). For example, fits of the control data estimate the contribution of the smallest events to be 13–15% ( Fig. 1b right) of all events that increases twofold after 20–25 min of antimycin-A treatment ( Fig. 2b ). Given this finding, we compared the frequency and amplitude of events smaller than −100 pA in recordings where antimycin-A was absent or included in the patch pipette ( Fig. 2c ). In control conditions, both mIPSC amplitude and frequency were similar throughout the duration of the experiment ( Fig. 2c , left). In contrast, however, small event frequency increased in a time-dependent manner in the presence of antimycin-A reaching a sustained maximum after 25 min ( Fig. 2c , right). 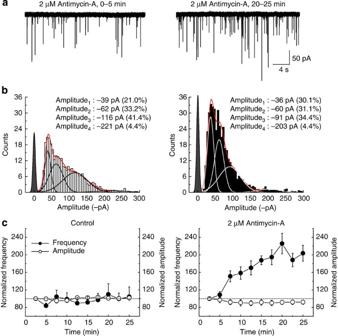Figure 2: Antimycin-A selectively enhances the occurrence of small amplitude inhibitory events. (a) mIPSCs from the same stellate cell (cell no. 111118p1) at two time periods in the presence of 2 μM antimycin-A. (b) Amplitude histograms comparing the data obtained at two time periods (0–5 min, left; 20–25 min, right) following the introduction of 2 μM antimycin-A (n=5). Averaged data have been fit with the sum of four Gaussian functions (red line) with individual Gaussians shown in either black (left panel) or white (right panel). (c) Summary plot showing how normalized small event (i.e.,<−100 pA) amplitude (open circle) or frequency (filled circle) changed with time in the presence (n=5) and absence (n=6) of antimycin-A. Error bars, s.e.m. For clarity, the lower (frequency) and upper (amplitude) error bars were removed in the control panel (left). Figure 2: Antimycin-A selectively enhances the occurrence of small amplitude inhibitory events. ( a ) mIPSCs from the same stellate cell (cell no. 111118p1) at two time periods in the presence of 2 μM antimycin-A. ( b ) Amplitude histograms comparing the data obtained at two time periods (0–5 min, left; 20–25 min, right) following the introduction of 2 μM antimycin-A ( n =5). Averaged data have been fit with the sum of four Gaussian functions (red line) with individual Gaussians shown in either black (left panel) or white (right panel). ( c ) Summary plot showing how normalized small event (i.e.,<−100 pA) amplitude (open circle) or frequency (filled circle) changed with time in the presence ( n =5) and absence ( n =6) of antimycin-A. Error bars, s.e.m. For clarity, the lower (frequency) and upper (amplitude) error bars were removed in the control panel (left). Full size image Interestingly, we also observed what appeared to be a small time-dependent reduction in the averaged amplitude of small events in the presence of antimycin-A ( Fig. 2c , right). For example, after 20–25 min, the event amplitude was −54.6±1.3 pA (mean±s.e.m.) which declined to 93.9±2.7% of the events observed at the start of the recording (i.e., −57.7±1.6 pA, n =5). As discussed later, this trend towards a reduction in event amplitude is not due to a shift in the chloride equilibrium potential ( Supplementary Fig. 1 ) but rather due to the recruitment of subunit-specific GABA A receptors. An important concern was whether the effects described above for antimycin-A would impact inhibitory transmission in current-clamped stellate cells recorded in physiological levels of internal chloride. To examine this, we evoked inhibitory events on stellate cells by placing a stimulating electrode in the molecular layer of the cerebellum and then compared recordings in the presence and absence of antimycin-A ( Fig. 3 ). Under these conditions, antimycin-A elicited a time-dependent increase in the extent to which inhibitory postsynaptic potentials hyperpolarized stellate cells ( Fig. 3a,b ). For example, in antimycin-A-treated cells, the peak hyperpolarization observed in the first 5 min increased to 132.5±7.7% (mean±s.e.m. ; n =5, P =0.035, paired, two-tailed Student’s t -test) which was not observed in control cells (e.g., 20–25 min: 93.7±10.8% of control 0–5 min, n =3, P =0.44, paired, two-tailed Student’s t -test; Fig. 3b ). To account for the duration of the evoked event, we also measured the area under the curve for each hyperpolarization. In antimycin-A-treated cells, the time course of hyperpolarization (i.e., area under the curve) was −140.7±51.9 mV*ms (mean±s.e.m., n =5) in the first 5 min which increased to −295.7±85.7 mV*ms at the 20–25 min period ( P =0.043, paired, two-tailed Student’s t -test; Fig. 3a,c ). This change in the duration of hyperpolarization was absent in control cells (mean±s.e.m., n =3; 0–5 min: −133.5±32.6 mV*ms; 20–25 min: −145.6±29.3 mV*ms). Taken together, these data suggest that antimycin-A is able to affect stellate cell excitability by strengthening the degree of inhibitory tone. 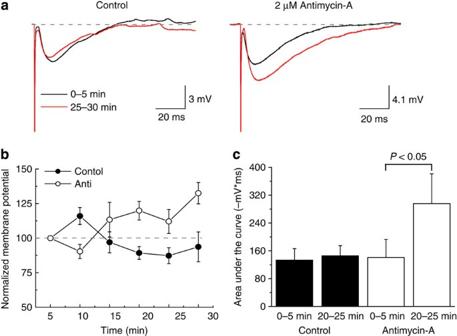Figure 3: Antimycin-A increases the amplitude of eIPSPs in the presence of physiological levels of chloride. (a) eIPSPs obtained in the presence (right) or absence (left) of 2 μM antimycin-A while cytosolic levels of chloride where maintained at physiological levels (i.e., [Cl−]I=4.1 mM). The black traces represent the average response during the first 5 min (i.e., 0–5 min). The red traces represent the average response during the last 5 min (i.e., 25–30 min). (b) Summary plot showing the change of normalized membrane potentials of eIPSPs in the presence (white circle;n=5) or absence (black circle;n=3) of 2 μM antimycin-A (Anti). (c) Summary bar graph comparing the change in the area under the curve for the control and 2 μM antimycin-A condition at two time points. When compared with the first 5 min (0–5 min), antimycin-A elicits a significant increase (P=0.043, paired two-tailed Student’st-test) in total area under the curve. Figure 3: Antimycin-A increases the amplitude of eIPSPs in the presence of physiological levels of chloride. ( a ) eIPSPs obtained in the presence (right) or absence (left) of 2 μM antimycin-A while cytosolic levels of chloride where maintained at physiological levels (i.e., [Cl − ] I =4.1 mM). The black traces represent the average response during the first 5 min (i.e., 0–5 min). The red traces represent the average response during the last 5 min (i.e., 25–30 min). ( b ) Summary plot showing the change of normalized membrane potentials of eIPSPs in the presence (white circle; n =5) or absence (black circle; n =3) of 2 μM antimycin-A (Anti). ( c ) Summary bar graph comparing the change in the area under the curve for the control and 2 μM antimycin-A condition at two time points. When compared with the first 5 min (0–5 min), antimycin-A elicits a significant increase ( P =0.043, paired two-tailed Student’s t -test) in total area under the curve. Full size image Antimycin-A affects mIPSC frequency by generating mROS Block of the electron transport chain impacts the cell in a number of ways; therefore, we performed several types of experiments to test whether the primary effect of antimycin-A was due to mROS. First, we imaged ROS levels by introducing the indicator dye, dichlorofluorescein (DCF) (see Methods), via the recording electrode while simultaneously measuring the frequency of mIPSCs in individual stellate cells ( Fig. 4 ). Analysis of these data revealed that the increase in mIPSC frequency elicited by antimycin-A was concomitant with an elevation in intracellular ROS ( Fig. 4b–d ). Although the increase in intracellular ROS was robust, it is likely an underestimate of the actual signal due to the time delay required to fill the cell with fluorescent indicators (red circles, Fig. 4c ). Second, the inclusion of the antioxidant, N-acetylcysteine (NAC; 1 mM), in the patch pipette attenuated the effect of antimycin-A on the frequency of small synaptic events ( Fig. 5a–c ). NAC contains a thiol group ( Fig. 5a , red lettering) that acts as an electron donor thereby conferring antioxidant effects by reducing the superoxide generated by antimycin-A. NAC (1 mM) alone had little effect on GABAergic transmission ( Fig. 5b ). Third, other mitochondrial uncouplers, myxothiazol (Myxo; 5 μM, Fig. 5a,c ) and rotenone (Rot; 2 μM, Fig. 5a,c ), mimicked the effect of antimycin-A by increasing the frequency ( Fig. 5c ) with a modest reduction in the averaged amplitude (e.g., Myxo; 20–25 min: 96.5±4.6% (mean±s.e.m.) of control, n =5) of small inhibitory synaptic events. Although myxothiazol is thought to bind to mitochondrial complex III, like antimycin-A [19] , it has been proposed to generate ROS through an effect on complex I, much like rotenone [21] , which may account for its apparently weaker effect on small event frequency ( Fig. 5c ). Finally, chemically derived ROS generated by the addition of the Fenton reaction (see Methods) in the patch pipette also elicited an increase in small GABAergic event frequency ( Fig. 5c ). Similar to antimycin-A, the Fenton reaction produced a steady increase in small event frequency over the first 15 min of the recordings but had a diminished effect over time (0.66±0.12 Hz (mean±s.e.m., n =5) at 10–15 min period to 0.45±0.07 Hz at 20–25 min, P =0.009, paired, two-tailed Student’s t -test). The return to basal levels of mIPSC frequency during prolonged exposure to the Fenton reaction was likely due to the time-dependent nature of the reaction. Furthermore, the modulating effects of Fenton-derived ROS may be impinged upon by the opposing effects of endogenous cytoplasmic antioxidants, such as glutathione, thus impeding ROS from reaching the synapse (i.e., the site of action). When taken together, these data suggest that mROS are responsible for the selective upregulation in frequency of small amplitude GABAergic synaptic events. 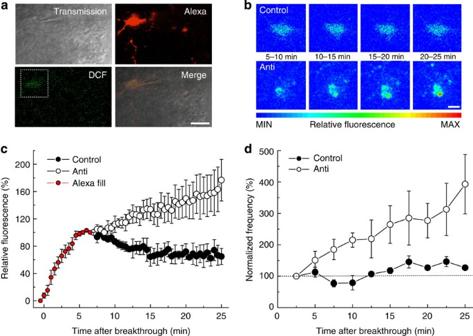Figure 4: Simultaneous fluorescence and electrophysiological measurements confirm that Antimycin-A increases intracellular ROS. (a) Representative scanning confocal images of a stellate cell loaded via the recording pipette with 100 μM Alexa 594 to assess the extent of cell filling and 100 μM H2DCF-DA (DCF) to measure increases in intracellular ROS. The inset is the area depicted in panelb(Control) at 2 min after breakthrough. Scale bar, 10 μm. (b) Example DCF images from two separate experiments in the absence (Control, cell no. 131010p1) and presence of antimycin-A (Anti, cell no. 131010p4) in the recording pipette. The images are displayed using a range indicator from blue, pixels with no fluorescence, to red, the maximum signal for any pixel over the course of an individual experiment. Scale bar, 5 μm (c) The time course of mean intracellular DCF fluorescence in control (n=3) and antimycin-A (n=4) experiments. Fluorescence was normalized based on the time it took to acquire a stable Alexa signal (5–7 min, Alexa fill). Error bars, s.e.m. (d) Normalized mean frequency time course of small amplitude mIPSCs (<−100 pA) recorded concomitantly from the same cells in (c). Error bars, s.e.m. Figure 4: Simultaneous fluorescence and electrophysiological measurements confirm that Antimycin-A increases intracellular ROS. ( a ) Representative scanning confocal images of a stellate cell loaded via the recording pipette with 100 μM Alexa 594 to assess the extent of cell filling and 100 μM H 2 DCF-DA (DCF) to measure increases in intracellular ROS. The inset is the area depicted in panel b (Control) at 2 min after breakthrough. Scale bar, 10 μm. ( b ) Example DCF images from two separate experiments in the absence (Control, cell no. 131010p1) and presence of antimycin-A (Anti, cell no. 131010p4) in the recording pipette. The images are displayed using a range indicator from blue, pixels with no fluorescence, to red, the maximum signal for any pixel over the course of an individual experiment. Scale bar, 5 μm ( c ) The time course of mean intracellular DCF fluorescence in control ( n =3) and antimycin-A ( n =4) experiments. Fluorescence was normalized based on the time it took to acquire a stable Alexa signal (5–7 min, Alexa fill). Error bars, s.e.m. ( d ) Normalized mean frequency time course of small amplitude mIPSCs (<−100 pA) recorded concomitantly from the same cells in ( c ). Error bars, s.e.m. 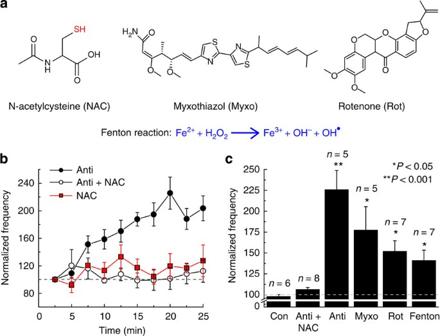Figure 5: Mitochondrial ROS increases the occurrence of small inhibitory events. (a) N-acetylcysteine (NAC), myxothiazol (Myxo), rotenone (Rot) structures as well as the Fenton reaction. The thiol group (highlighted in red) of NAC confers antioxidant properties. (b) Summary plot of antagonistic effect of NAC on the increase in small event frequency elicited by antimycin-A (2 μM Anti,n=5; 2 μM Anti+1 mM NAC,n=8 and 1 mM NAC,n=5). Error bars, s.e.m. (c) Summary bar graph comparing the normalized small event frequency (i.e.,<−100 pA) in different experimental conditions. When compared with control conditions (Con), the increase in event frequency observed with 2 μM antimycin-A (n=5,P=0.0002), 5 μM myxothiazol (n=5,P=0.0123), 2 μM rotenone (n=7,P=0.0028) and the Fenton reaction (n=7,P=0.0072) all reached statistical significance. All statistics were determined using an unpaired, two-tailed Student’st-test with the Bonferroni correction. Error bars, s.e.m. Full size image Figure 5: Mitochondrial ROS increases the occurrence of small inhibitory events. ( a ) N-acetylcysteine (NAC), myxothiazol (Myxo), rotenone (Rot) structures as well as the Fenton reaction. The thiol group (highlighted in red) of NAC confers antioxidant properties. ( b ) Summary plot of antagonistic effect of NAC on the increase in small event frequency elicited by antimycin-A (2 μM Anti, n =5; 2 μM Anti+1 mM NAC, n =8 and 1 mM NAC, n =5). Error bars, s.e.m. ( c ) Summary bar graph comparing the normalized small event frequency (i.e.,<−100 pA) in different experimental conditions. When compared with control conditions (Con), the increase in event frequency observed with 2 μM antimycin-A ( n =5, P =0.0002), 5 μM myxothiazol ( n =5, P =0.0123), 2 μM rotenone ( n =7, P =0.0028) and the Fenton reaction ( n =7, P =0.0072) all reached statistical significance. All statistics were determined using an unpaired, two-tailed Student’s t -test with the Bonferroni correction. Error bars, s.e.m. Full size image mROS promotes the occurrence of slow-decaying mIPSCs A change in the frequency of synaptic activity, as observed with antimycin-A, is usually indicative of a presynaptic mechanism [22] . However, a comparison of event decay kinetics observed in the presence and absence of antimycin-A suggests that mROS may instead be primarily acting at a postsynaptic site. To perform the comparison, synaptic events were each fitted with a single exponential function and this value was plotted with respect to the peak response amplitude ( Fig. 6a ). In the absence of antimycin-A, most synaptic events (open circles) had a decay time constant of 10.16±0.17 ms (mean±s.e.m. ; n =6) irrespective of the peak amplitude ( Fig. 6a ). We did, however, observe a few events with slower decay kinetics, which were more readily identified in fits of the distribution in decay kinetics ( Fig. 6b , upper panel). Of note, mIPSCs with slower decay kinetics were usually associated with smaller peak responses ( Fig. 6a ). 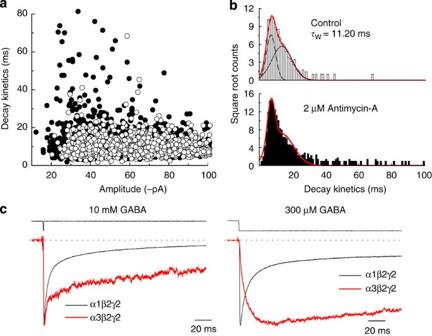Figure 6: Slow mIPSCs and recombinant α3-GABAAreceptors have similar kinetics. (a) Plot of mIPSC amplitude and decay kinetics of small amplitude (i.e.,<−100 pA) events observed in control (white circles,n=6) or 2 μM antimycin-A (black circles,n=5) conditions. (b, upper panel) Histograms showing the distribution of mIPSC decay kinetics fit with the sum of two Gaussian functions (red line). Individual Gaussians are shown in black. (b, lower panel) Similar plot of the distribution of decay kinetics observed in the presence of antimycin-A. The Gaussian fit (red line) from the upper panel has been scaled onto the data to identify the many more slow-decaying mIPSCs observed with antimycin-A exposure. (c) Overlay of typical membrane currents elicited by short 1 ms (left) or long 250 ms (right) applications of 10 mM or 300 μM GABA acting on recombinant α1β2γ2 (black line, patch no. 130322p7) or α3β2γ2 (red line, patch no. 130308p3) receptors. Response amplitudes have been normalized to allow a comparison of decay kinetics. Figure 6: Slow mIPSCs and recombinant α3-GABA A receptors have similar kinetics. ( a ) Plot of mIPSC amplitude and decay kinetics of small amplitude (i.e.,<−100 pA) events observed in control (white circles, n =6) or 2 μM antimycin-A (black circles, n =5) conditions. ( b , upper panel) Histograms showing the distribution of mIPSC decay kinetics fit with the sum of two Gaussian functions (red line). Individual Gaussians are shown in black. ( b , lower panel) Similar plot of the distribution of decay kinetics observed in the presence of antimycin-A. The Gaussian fit (red line) from the upper panel has been scaled onto the data to identify the many more slow-decaying mIPSCs observed with antimycin-A exposure. ( c ) Overlay of typical membrane currents elicited by short 1 ms (left) or long 250 ms (right) applications of 10 mM or 300 μM GABA acting on recombinant α1β2γ2 (black line, patch no. 130322p7) or α3β2γ2 (red line, patch no. 130308p3) receptors. Response amplitudes have been normalized to allow a comparison of decay kinetics. Full size image Antimycin-A affected synaptic activity in two ways. First, many more small amplitude events were observed with decay kinetics slower than 30 ms ( Fig. 6a,b , lower panel). In the presence of antimycin-A, the number of events with slow decay kinetics increased about threefold, from ~0.7% (7/967 events) in control conditions to about 3% (51/1665 events). Second, antimycin-A substantially increased the number of events with amplitudes ≤ −30 pA (antimycin-A: 208 events or 12.5% of all small events; control: 34 events or 3.5% of all small events; Fig. 6a ). This observation explains the modest reduction of the averaged response amplitude elicited by antimycin-A ( Fig. 2c , right panel). It is unlikely that the occurrence of small amplitude, slow-decaying synaptic events was the result of poorly voltage-clamped synapses on distal dendritic branches, since their occurrence in ROS-generated solutions (i.e., antimycin-A, myxothiazol, rotenone and the Fenton reaction) was not associated with any change in the cells’ biophysical properties. Consequently, we concluded that the appearance of small amplitude, slow-decaying mIPSCs has a biological origin and that mROS affect inhibitory transmission mainly through a postsynaptic mechanism. Given the greater occurrence of small amplitude events with slow decay kinetics, we thus postulated that ROS may be strengthening inhibitory transmission by recruiting GABA A receptors possibly from extrasynaptic sites [23] , [24] . The slowing observed in decay kinetics would, in this case, correspond to recruited receptors responding to the neurotransmitter gradient emanating from inhibitory synapses. The subunit composition of extrasynaptic GABA A receptors expressed by stellate cells is not known, although it is most likely assembled from α1-(refs 15 , 16 ) and/or α3-containing receptors [17] , [18] . Therefore, we next determined whether the kinetic properties of recombinant α1- and/or α3-containing receptors matched that of the slow-decaying synaptic events observed during antimycin-A treatment. To do this, we co-expressed α1- or α3 subunits with β2 and γ2 subunits in mammalian cells from which we excised outside-out patches ( Fig. 6c , Supplementary Table 1 ). Brief (1 ms) applications of 10 mM γ-aminobutyric acid (GABA) to excised patches were used to mimic the response elicited by neurotransmitter released into the synaptic cleft, whereas long (250 ms) applications of 300 μM GABA were used to mimic the concentration profile of extrasynaptic GABA (see Barberis et al. [25] for details on the synaptic/extrasynaptic concentration profile of GABA). Using this approach, the decay kinetics of α1-containing GABA A receptors were dominated by a fast component of ~3 ms when activated by either 300 μM or 10 mM GABA ( Fig. 6c , Supplementary Table 1 ), which does not match the slower kinetics of synaptic events observed in antimycin-A. In contrast, α3-containing receptors decayed at least an order of magnitude slower in response to both high and low GABA concentrations ( Fig. 6c , Supplementary Table 1 ), which was more in line with the kinetic behaviour of synaptic events. In keeping with this, we concluded that the slowing of decay kinetics was not due to a direct pharmacological action on α3-containing GABA A receptors since application of antimycin-A to outside-out patches (external or cytoplasmic side of the membrane) did not affect their gating properties ( Supplementary Fig. 2 ). Taken together, these data suggest that the increase in occurrence of slow-decaying events is consistent with the recruitment of α3-containing GABA A receptors into inhibitory synapses. To test this hypothesis directly, we next examined the effect of antimycin-A on GABAergic currents recorded in mice lacking either α1 or α3 GABA A receptor subunits. mROS have no effect on mIPSC frequency in α3-KO mice We started with α3-knockout (KO) mice since the recombinant data suggested an important role for this subunit in mROS-mediated changes of GABAergic synapses. Similar to the wild-type mice, mIPSCs of stellate cells in α3-KO mice varied in amplitude between −20 pA and −300 pA, although a greater proportion of mIPSCs were of small amplitude ( Fig. 7a,b ). Unlike wild-type mice, however, the inclusion of antimycin-A in the patch electrode had no significant effect on small mIPSC frequency ( Fig. 7c ). For example, the frequency observed during the final 5 min was 0.85±0.08 Hz (mean±s.e.m.) which was similar to the frequency of 0.90±0.1 Hz observed during the first 5 min ( n =5, P =0.35, paired, two-tailed Student’s t -test). Likewise, antimycin-A did not promote the occurrence of events with slow decay kinetics ( Fig. 7d ). The total number of events with decay kinetics >30 ms was 1.1% (5/466 events) for the first 5 min and 0.91% (5/549 events) in the last 5 min. The average decay time constant increased significantly in the last 5 min (10.03±0.2 ms; mean±s.e.m.) when compared with the first 5 min (7.23±0.2 ms; n =5, P <0.0001, paired, two-tailed Student’s t -test). It is not clear why there is a slowing in decay kinetics, although it is possible that antimycin-A may also act on α2-containing GABA A receptors, which have been reported to be expressed by stellate cells [17] . In terms of small event amplitudes, antimycin-A had no effect on their overall occurrence (i.e.,<−30 pA; 0–5 min: 37/466 or 7.9%; 20–25 min: 46/549 or 8.4%). Taken together, these data suggest that the ROS-mediated increase in small amplitude, slow-decaying mIPSCs is absent in stellate cells lacking α3-containing GABA A receptors. 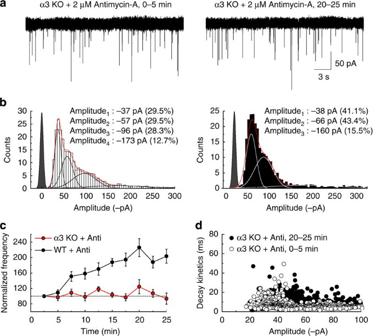Figure 7: Mitochondrial ROS do not strengthen inhibitory synapses lacking the α3 subunit. (a) mIPSCs recorded from the same stellate cell (cell no. 121130p1) in an α3-KO mouse during internal perfusion with 2 μM antimycin-A. (b) Amplitude histograms comparing data (n=5) obtained at two time periods (i.e., 0–5 min, left; 20–25 min, right). Pooled data has been fit with the sum of 3–4 Gaussian functions (red line) with individual Gaussians shown in either black (left panel) or white (right panel). (c) Summary plot comparing the effect of antimycin-A on small amplitude event frequency in wild-type (n=6) and α3-KO (n=5) mice. Error bars, s.e.m. (d) Scatter plot comparing decay kinetics and mIPSC amplitudes at two time points in stellate cells from α3-KO mice (n=5). Figure 7: Mitochondrial ROS do not strengthen inhibitory synapses lacking the α3 subunit. ( a ) mIPSCs recorded from the same stellate cell (cell no. 121130p1) in an α3-KO mouse during internal perfusion with 2 μM antimycin-A. ( b ) Amplitude histograms comparing data ( n =5) obtained at two time periods (i.e., 0–5 min, left; 20–25 min, right). Pooled data has been fit with the sum of 3–4 Gaussian functions (red line) with individual Gaussians shown in either black (left panel) or white (right panel). ( c ) Summary plot comparing the effect of antimycin-A on small amplitude event frequency in wild-type ( n =6) and α3-KO ( n =5) mice. Error bars, s.e.m. ( d ) Scatter plot comparing decay kinetics and mIPSC amplitudes at two time points in stellate cells from α3-KO mice ( n =5). Full size image mROS increase mIPSC frequency in α1-KO mice Inhibitory synapses of stellate cells in α1-KO mice differed from their wild-type counterpart in several important ways. First, all recorded mIPSCs in the α1-KO mice were much smaller in amplitude averaging about −30.6±0.34 pA (mean±s.e.m. ; n =5) compared with −104.1±0.73 pA of wild-type stellate cells ( Fig. 8a ). In fact, few synaptic responses ever surpassed −100 pA in amplitude consistent with a previous study [18] . Second, the decay kinetics of small mIPSCs in α1-KO mice were much slower ( Fig. 8a ) averaging about 20.2±0.60 ms (mean±s.e.m. ; n =5) compared with 10.16±0.17 ms (mean±s.e.m. ; n =6) in wild-type mice. A comparison of response amplitude versus decay kinetics of small mIPSCs observed in wild-type (open circles) and α1-lacking (black circles) mice revealed that the profile of inhibitory events in α1-KO mice were reminiscent of the small amplitude, slow-decaying responses observed in wild-type mice following antimycin-A treatment ( Fig. 8b ). Third and finally, mIPSC frequency in α1-lacking mice was lower at 0.52±0.05 Hz (mean±s.e.m. ; n =5); an observation that might be expected given the preponderance of α1-containing GABA A receptors in stellate cells. Taken together, these observations suggest upregulation of the α3 subunit in the cerebellum of α1-KO mice, as suggested previously [26] and shown directly in Supplementary Fig. 3 . 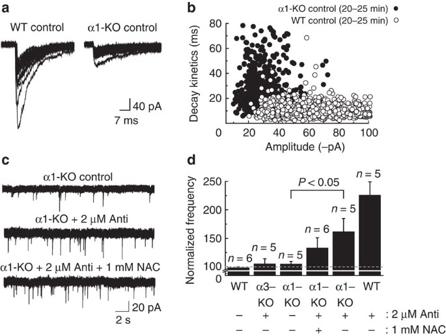Figure 8: Mitochondrial ROS increase mIPSC frequency in stellate cells lacking the α1-subunit. (a) Comparison of 15 randomly selected mIPSCs recorded in wild-type (left) and α1-KO (right) stellate cells. (b) Scatter plot comparing decay kinetics and amplitudes of mIPSCs from stellate cells in wild-type (n=6) and α1-KO mice (n=5). (c) Representative mIPSCs showing the effect of internal perfusion with 2 μM antimycin-A (top trace, cell no. 121025p2; middle trace, cell no. 121016p1 and bottom trace, cell no. 121206p1). (d) Bar graph summarizing the effect of antimycin-A on mIPSC frequency in wild-type and α1-KO cells. Statistics were determined using an unpaired, two-tailed Student’st-test;P=0.0484. Error bars, s.e.m. Figure 8: Mitochondrial ROS increase mIPSC frequency in stellate cells lacking the α1-subunit. ( a ) Comparison of 15 randomly selected mIPSCs recorded in wild-type (left) and α1-KO (right) stellate cells. ( b ) Scatter plot comparing decay kinetics and amplitudes of mIPSCs from stellate cells in wild-type ( n =6) and α1-KO mice ( n =5). ( c ) Representative mIPSCs showing the effect of internal perfusion with 2 μM antimycin-A (top trace, cell no. 121025p2; middle trace, cell no. 121016p1 and bottom trace, cell no. 121206p1). ( d ) Bar graph summarizing the effect of antimycin-A on mIPSC frequency in wild-type and α1-KO cells. Statistics were determined using an unpaired, two-tailed Student’s t -test; P =0.0484. Error bars, s.e.m. Full size image As predicted from the role of α3-containing GABA A receptors in wild-type mice, the frequency of mIPSCs in stellate cells of α1-KO mice increased in a time-dependent manner when antimycin-A was included in the patch pipette ( Fig. 8c,d ). Antimycin-A increased event frequency from 0.63±0.1 Hz (mean±s.e.m.) within the first 5 min to 0.85±0.1 Hz in the last 5 min ( n =5, P =3.24 × 10 −5 , paired, two-tailed Student’s t -test) of the recording corresponding to a normalized maximal peak increase of 68.6±28.7% ( Fig. 8c,d ). We concluded that antimycin-A regulated mIPSC frequency by generating mROS since the effect of the mitochondrial uncoupler on event frequency ( Fig. 8c,d ) and amplitude ( Supplementary Fig. 4 ) was attenuated by 1 mM NAC. Finally, in the last 5 min, antimycin-A increased the occurrence of slow-decaying mIPSCs with time constants greater than 30 ms (24%, 324 events). Thus, these data suggest that the ROS-mediated increase in small amplitude, slow-decaying mIPSCs occurs through the recruitment of α3-containing GABA A receptors. It is interesting that antimycin-A increased event frequency in α1-lacking stellate cells less than in wild-type neurons ( Fig. 8d ). Since wild-type inhibitory synapses mainly possess α1-containing GABA A receptors [15] , [17] , we reasoned that antimycin-A would be able to recruit more α3-containing GABA A receptors into these synapses. This explanation would explain the apparently weaker effect of mROS on α1-lacking stellate cells which, importantly, could be tested experimentally. Specifically, we hypothesized that mROS should increase not only the inhibitory event frequency in α1-lacking stellate cells but also their amplitude as more α3-containing GABA A receptors are recruited into the synapse. mROS also increase mIPSC amplitude in α1-KO mice As expected, neither the mIPSC frequency nor amplitude changed in control recordings of stellate cells lacking the α1-subunit ( Fig. 9a , left panel). However, in antimycin-A-treated cells, the frequency of inhibitory events increased suggesting that the α1-subunit does not play a major role ( Fig. 9a , right panel). The total event frequency during the first 5 min significantly increased after 20–25 min ( Figs 8d , 9a , right). This increase was also observed by fitting the amplitude distributions ( Fig. 9b ). Interestingly, this analysis also uncovered an appreciable increase in the amplitude of mIPSCs ( Fig. 9b , right panel). Fits of the amplitude distributions taken from the last 5 min of control α1-KO mice revealed that mIPSCs were best fit by the sum of two Gaussian components (−23 pA (43.1%) and −31 pA (56.9%)). However, after 20–25 min of antimycin treatment, data were best fit by four Gaussian components (−21 pA (41.5%), −32 pA (36.8%), −50 pA (15.0%) and −88 pA (6.7%)), where a sizeable proportion of all events (about 22%) exhibited amplitudes that were two- to threefold larger than any mIPSCs observed during the α1-KO-control condition. Taken together, these data demonstrate that antimycin-A increases both the frequency and amplitude of mIPSCs in stellate cells lacking the α1-subunit by recruiting α3-containing GABA A receptors to synaptic sites. Interestingly, when we repeated these experiments in younger wild-type mice (i.e., P10–12), where α3- and not α1-containing GABA A receptors dominate the synaptic response (see Vicini et al. [18] ), antimycin-A increased event frequency, as expected, but did not increase mIPSC amplitude ( Fig. 10 ) suggesting that the rules regulating synaptic strength are distinct in developing and mature stellate cells. 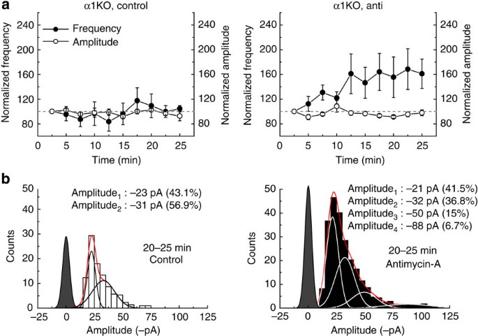Figure 9: ROS increase mIPSC frequency and amplitude in α1-KO mice. (a,b) Summary plots comparing mIPSC frequency and amplitude (i.e.,<−100 pA) in α1-KO mice in the presence (right,n=5) and absence (left,n=5) of 2 μM antimycin-A. Error bars, s.e.m. (b) Amplitude distributions of mIPSCs observed during the last 5 min (i.e., 20–25 min) of stellate cell recordings from α1-KO mice both in the presence (right) and absence (left) of 2 μM antimycin-A. Averaged data have been fit with the sum of two or four Gaussian functions (red line) with individual Gaussians shown in either black (left panel) or white (right panel). Figure 9: ROS increase mIPSC frequency and amplitude in α1-KO mice. ( a , b ) Summary plots comparing mIPSC frequency and amplitude (i.e.,<−100 pA) in α1-KO mice in the presence (right, n =5) and absence (left, n =5) of 2 μM antimycin-A. Error bars, s.e.m. ( b ) Amplitude distributions of mIPSCs observed during the last 5 min (i.e., 20–25 min) of stellate cell recordings from α1-KO mice both in the presence (right) and absence (left) of 2 μM antimycin-A. Averaged data have been fit with the sum of two or four Gaussian functions (red line) with individual Gaussians shown in either black (left panel) or white (right panel). 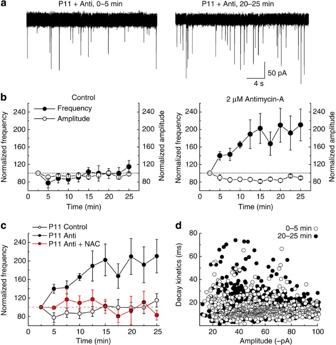Figure 10: Antimycin-A increases the occurrence of small inhibitory events during early stellate cell development. (a) mIPSCs from the same stellate cell (cell no. 138050p3) at two time periods in the presence of 2 μM antimycin-A (Anti). (b) Summary plot showing how normalized small event (i.e.,<−100 pA) amplitude (open circle) or frequency (filled circle) changed with time in the presence (n=7) and absence (n=8) of antimycin-A. Error bars, s.e.m. (c) Summary plot showing the time course of the small mIPSC frequency increase elicited by 2 μM antimycin-A (Anti, black circle) and the antagonistic effect of NAC (red circle,n=7). The control condition (white circle) did not change over time. Error bars, s.e.m. (d) Plot of mIPSC amplitude and decay kinetics of small amplitude (i.e.,<−100 pA) events observed in the first (i.e., 0–5 min, white circles) and last (i.e., 20–25 min, black circles) 5 min of young (P11) mice in the presence of 2 μM antimycin-A. Full size image Figure 10: Antimycin-A increases the occurrence of small inhibitory events during early stellate cell development. ( a ) mIPSCs from the same stellate cell (cell no. 138050p3) at two time periods in the presence of 2 μM antimycin-A (Anti). ( b ) Summary plot showing how normalized small event (i.e.,<−100 pA) amplitude (open circle) or frequency (filled circle) changed with time in the presence ( n =7) and absence ( n =8) of antimycin-A. Error bars, s.e.m. ( c ) Summary plot showing the time course of the small mIPSC frequency increase elicited by 2 μM antimycin-A (Anti, black circle) and the antagonistic effect of NAC (red circle, n =7). The control condition (white circle) did not change over time. Error bars, s.e.m. ( d ) Plot of mIPSC amplitude and decay kinetics of small amplitude (i.e.,<−100 pA) events observed in the first (i.e., 0–5 min, white circles) and last (i.e., 20–25 min, black circles) 5 min of young (P11) mice in the presence of 2 μM antimycin-A. Full size image The present study advances our understanding of inhibitory GABAergic synapses in two important ways. First, we show that cellular metabolism regulates the strength of inhibitory transmission by generating mROS. As discussed below, the traditional view that mROS are primarily involved in oxidative stress has broadened to encompass a more physiological role for these versatile signalling molecules [27] . Second, strengthening of stellate cell inhibitory synapses occurs through a mechanism that is selective for the recruitment of α3-containing GABA A receptors. Curiously, mROS have no apparent effect on α1-receptors which are the predominant GABA A receptor present at stellate cell inhibitory synapses. This apparent discrepancy can be explained if α3 receptors are recruited into synaptic sites that are distinct from α1 receptors. Given this, our data are consistent with the idea that α3-containing GABA A receptors occupy synaptic sites which are either entirely devoid of any GABA A receptor, reminiscent of silent glutamatergic [28] or GABAergic [29] synapses, and/or contain a small number of α3-containing receptors. The generation of mROS has been traditionally linked to the cellular damage that accompanies chronic disease states such as diabetes [30] , cancer [31] and neurodegenerative conditions such as Alzheimer’s disease and Parkinsonism [32] . Given this, it might be concluded that our experiments using antimycin-A are more in line with these chronic disease states. However, recent work in the striatum suggests that the elevation in ROS elicited by mitochondrial uncouplers and physiological stimuli can be quite comparable [33] . Consequently, our findings may point to a more physiological role for mROS as already described for the innate immune response as well as the control of embryonic stem cell differentiation [27] . Exactly how mROS are elevated in inhibitory stellate cells awaits future study. However, given the emerging view that mROS lay at the heart of an important signalling hub [27] , it is likely that numerous biochemical pathways converge on stellate cell synapses to elevate mROS. We were initially surprised that mROS regulated α3-containing receptors with no apparent effect on α1-receptors. This observation can be explained in one of two ways. First, α1- and α3- containing GABA A receptors may be recruited to morphologically distinct stellate cell inhibitory synapses. In fact, subunit-specific synaptic segregation is not unusual for the cerebellum [34] . Granule cells, for example, form inhibitory synapses with Golgi cells which contain primarily α1β2/3γ2 (with some α6β2/3γ2 receptors), whereas mossy fibre to granule cell synapses contain only α6β2/3γ2 receptors [35] . In keeping with this, stellate cells are innervated by other cell types that include other stellate cells and basket cells of the molecular layer as well as Lugaro cells and globular cells, which are located beneath the Purkinje cell layer [34] , [36] . Consequently, it is possible that α1- and α3- containing GABA A receptors are targeted to synapses that are formed with different presynaptic partners. Second, α1- and α3- containing GABA A receptors may still share the same presynaptic terminal but are activated by neurotransmitter released from functionally-distinct active zones. In support of this, serial electron micrographs of inhibitory stellate cell synapses reveal their unusual architecture that places different active zones of the same presynaptic terminal in discrete locations [12] . This arrangement may allow α1- and α3- containing GABA A receptors to act in the distinct manner reported in our study. The physiological value of segregating GABA A receptors at stellate cell inhibitory synapses is not yet clear, although it is possible that the different kinetic properties of α1- and α3-receptors may allow neuronal excitability to be finely controlled. In α1-lacking mice, the situation is similar but with the difference that α3-containing GABA receptors are now present to a greater extent at inhibitory synapses (see Fig. 8a and Supplementary Fig. 3 ). Given this, the relative increase in event frequency elicited by antimycin-A would be expected to be less, as we have observed, since many synapses already contain α3-receptors. Moreover, since the event amplitude increases in α1-lacking mice, this observation suggests that α3-containing GABA receptors are recruited to sites already containing α3-receptors. In principle, a number of mechanisms may account for the increase in occurrence of α3-containing GABA A receptors with mROS which include lateral relocation of extrasynaptic receptors into inhibitory synapses [23] , [37] , exocytotic insertion of synaptic GABA A receptors and/or mROS-directed increase in GABA A receptor open-channel probability. More work is required to delineate between these possibilities; however, our data are consistent with the recruitment of extrasynaptic α3-containing receptors. In agreement with this, lateral movement of extrasynaptic receptors has been proposed to be the dominating mechanism that strengthens GABAergic synapses [23] , [24] , [37] . Moreover, the time frame of lateral diffusion is also consistent with the rates of mROS modulation described in the present study. Lateral relocation is dependent upon the diffusion rate of a receptor which interestingly, is higher for extrasynaptic GABA A receptors [23] , [37] , [38] , [39] . Finally, the occurrence of small amplitude, slow-decaying synaptic events elicited by mROS is also consistent with the lateral movement of α3-containing GABA A receptors, which would be expected to have these properties in response to low GABA concentrations. Clearly, more work is still required to understand how the generation of ROS in the mitochondria triggers the events that lead to the strengthening of inhibitory synapses of cerebellar stellate cells. Moreover, it would be important in future studies to examine if this effect of mROS is common to all inhibitory synapses. Animals Homozygous GABA A receptor α1-KO mice were generated on a mixed C57BL/6J-129Sv/SvJ background at the University of Pittsburgh (Pittsburgh, PA, USA) [18] and bred at the University of Zurich. Wild-type and α3-KO mice were maintained on a C57BL/6J background (B6.129 1-Gabra3tm2Uru/Uru) [40] and also bred at the University of Zurich. As the α3 subunit gene is located on the X chromosome, mutant mice were either hemizygote male or homozygote female obtained from heterozygous/hemizygous or α3-KO breeding pairs. Wild-type mice with a C57BL/6J background were obtained from Jackson Laboratories (Bar Harbor, ME, USA) and maintained as a breeding colony at McGill University. All animals were genotyped by PCR analysis of tail biopsies. Mutant mice were born at the expected Mendelian ratio and the mutant phenotypes were maintained across generations. Mice (WT and α1-KO: male and female, α3-KO: males only) used for the experiments ranged from 15 to 28 days old (P15–28; mean±s.e.m. age: P22±1, n =46) or 10–12 days old (P10–12; mean±s.e.m. age: P11±1, n =7; only for Fig. 10 ). All experiments have been approved by the local authorities and were performed in accordance with the guidelines of the Canadian Council on Animal Care and European Community Council Directive 86/609/EEC and were approved by the Animal Care Committee of McGill University (Protocol Number: 4564) or the Cantonal Veterinary Office of Zurich. Cerebellum slice preparation Mice were anaesthetized with isoflurane and immediately decapitated. The cerebellum was rapidly removed from the whole brain while submerged in oxygenated (95% O 2 , 5% CO 2 ) ice-cold cutting solution. Cutting solution contained (in mM): 235 sucrose, 2.5 KCl, 1.25 NaH 2 PO 4 , 28 NaHCO 3 , 0.5 CaCl 2 , 7 MgSO 4 and 28 D-glucose (pH of 7.4; 305–315 mOsmol l −1 ). The tissue was maintained in ice-cold solution while sagittal slices of cerebellum (250–300 μm) were cut using a vibrating tissue slicer (Leica VT100S, Leica Instruments, Nussloch, Germany). The slices were transferred to oxygenated, room temperature (20–23 °C) artificial cerebrospinal fluid (aCSF) for at least 1 h before recordings. aCSF contained (in mM): 125 NaCl, 2.5 KCl, 1.25 NaH 2 PO 4 , 26 NaHCO 3 , 2 CaCl 2 , 1 MgSO 4 and 25 D-glucose (pH of 7.4; 305–315 mOsmol l −1 ). Cell culture and transfection Human embryonic kidney (HEK) 293T/17 cells (ATCC CRL-11268, Manassas, VA, USA) were maintained at 70–80% confluency in minimal essential medium with Earle’s salts, 2 m M glutamine and 10% fetal bovine serum. After plating at low density (2 × 10 4 cells per ml) on 35 mm plastic dishes coated with poly-D-lysine, cells were transfected with the complementary DNAs (cDNAs) encoding the GABA A receptor subunits in a 1:1:2 ratio (α1:β2:γ2), using the calcium phosphate technique. All GABA A receptor subunits used were of human sequences, except the α3 subunit, which was of the rat sequence. The cDNA for enhanced green fluorescent protein was routinely co-transfected (0.1 μg per dish) to identify transfected cells. Electrophysiology Slice experiments were performed on an Olympus BX51 upright microscope (Olympus, Southall, UK) equipped with differential interference contrast/infrared optics. Whole-cell patch-clamp recordings were made from stellate cells which were distinguished from misplaced or migrating granule, glial or basket cells by their small soma diameter (8–9 μm) and location in the outer two-thirds of the molecular layer. Patch pipettes were prepared from thick-walled borosilicate glass (GC150F-10, OD 1.5 mm, ID 0.86 mm; Harvard Apparatus Ltd, Kent, UK) and had open tip resistances of 3–8 MΩ when filled with an intracellular solution that contained (in mM): 140 CsCl, 4 NaCl, 0.5 CaCl 2 , 10 HEPES, 5 EGTA, 2 Mg-ATP, 2 QX314 to block voltage-activated Na + channels and 0.5 mg ml −1 Lucifer Yellow as a post hoc dye indicator (pH 7.4 with CsOH, 300–310 mOsmol l −1 ). Recordings were made with a Multiclamp 700A amplifier (Molecular Devices, Sunnyvale, CA, USA) at a holding potential of −60 mV. Series resistance and whole-cell capacitance were estimated by cancelling the fast current transients evoked at the onset and offset of brief (10–20 ms) 5 mV voltage-command steps. Series resistance during postsynaptic whole-cell recording (10–35 MΩ) was compensated between 40 and 65% and checked for stability throughout the experiments (>20% tolerance). The capacitance of the stellate cells was in the range of 6–11 pF. The bath was continuously perfused at room temperature (22–23 °C) with aCSF at a rate of 1–2 ml min −1 . mIPSCs were recorded in the presence of TTX (1 μM). Currents were filtered at 5 kHz with either a four-pole or eight-pole low-pass Bessel filter (Frequency Devices, Haverhill, MA, USA) and digitized at 25 kHz with a Digidata 1322A data acquisition board and Clampex9 (Molecular Devices) software. For extracellular stimulation, thin-walled borosilicate glass electrodes (OD 1.65 mm, ID 1.15 mm; King Precision Glass Inc., Claremont, CA, USA) were used with a tip current of <3 MΩ when filled with aCSF. The intracellular solution used for evoked potentials contained (in mM): 126 K-Gluconate, 0.05 CaCl 2 , 0.15 K 4 BAPTA, 4 NaCl, 1 MgSO 4 , 15 D-Glucose, 5 HEPES, 3 Mg-ATP, 0.1 NaGTP, 2 QX314 (pH 7.4 with KOH, 300–310 mOsmol l −1 ). The ground electrode for the stimulation circuit was made with a platinum wire wrapped around the stimulation electrode. The stimulating electrode was positioned in the molecular layer at or just beneath the slice surface. Voltage pulses (1–25 V in amplitude, 200–400 ms in duration) were applied at low frequency stimulation (0.05–0.03 Hz) through the stimulating electrode. To minimize variability between responses, the stimulating electrode was positioned between 50 and 100 μm away from the cell of interest. The voltage that was used during each experiment was the lowest voltage intensity obtained that elicited the maximal eIPSPs response. Experiments were also performed at room temperature on recombinant GABA A receptors 24–48 h after cDNA transfection. GABA (Sigma-Aldrich, St Louis, MO, USA) was dissolved in external solution containing (in mM): 150 NaCl, 5 HEPES, 2 MgCl 2 and 1 CaCl 2 . Internal pipette solution contained (in mM): 150 KCl, 5 EGTA, 1 MgCl 2 and 2 Mg-ATP. The pH and osmotic pressure of internal and external solutions were adjusted to 7.3–7.4 and 300 mOsm l −1 , respectively. All recordings were performed with an Axopatch 200B amplifier (Molecular Devices) using thin-walled borosilicate glass pipettes (2–5 MΩ) coated with dental wax to reduce electrical noise. Control and agonist solutions were rapidly applied to outside-out patches excised from transfected HEK 239T/17 cells using a piezoelectric stack (Physik Instrumente, Karlsruhe/Palmbach, Germany). Solution exchange (10–90% rise-time=150–250 μs) was determined by measuring the liquid junction current (or exchange current) between the control and external solution containing 10% additional NaCl. Current records were filtered at 5 kHz, digitized at 25 kHz and series resistances (3–10 MΩ) were compensated by 95%. All recordings were performed at a holding potential of −60 mV. Data acquisition were performed using pClamp10 software (Molecular Devices). Curve fitting and figure preparation of all electrophysiology data were performed with Origin 7.0 (OriginLab, Northampton, MA, USA), Microsoft Excel, Clampfit 10 (Molecular Devices) and the Strathclyde Electrophysiology WinWCP and WinEDR (John Dempster, Glasgow, UK) software. Analysis of mIPSC events mIPSCs were detected using WinEDR software with a detection threshold of four times the mean root square noise level. The accuracy of detection was visually confirmed for each recording. Only cells exhibiting mIPSC frequency of greater than 0.2 Hz were used for analysis. Amplitude distributions were fit with the sum of 2–4 Gaussian functions with the singular form of: y =(Ai/wi*sqrt( π /2)))*exp(−2*((x−xci)/wi)2), where A is the area, xc is the centre of the peak and w is the error associated with the peak. The decay phase of mIPSCs was fit with a single exponential curve and both rise and decay phase were fitted between 10 and 90% of the peak amplitude. Data are expressed as mean±s.e.m. ; P -values represent the results of paired or unpaired, two-tailed Student’s t -tests. A P -value of less than 0.05 was considered statistically significant. All data are from at least two different animals. Intracellular ROS fluorescence Scanning confocal images were collected on a Zeiss Axioexaminer microscope (Carl Zeiss Microscopy Jena GmbH, Jena, Germany) in the McGill University Life Sciences Complex Advanced BioImaging Facility. mIPSCs were simultaneously recorded on a HEKA EPC10 amplifier (HEKA Electronik Dr Schulze GmbH, Lambrecht/Pfalz, Germany) and visualized with HEKA Patchmaster software. Solutions for recording stellate cell mIPSCs were used as above except the internal solution included Alexa 594 (100 μM; Life Technologies Inc., Burlington, ON, Canada) to report the extent of indicator filling and CM-H 2 DCF-DA (100 μM; Life Technologies Inc.) to report the relative increase in intracellular ROS [41] . Pairs of images were collected every 30 s, to reduce potential photo-oxidation of the ROS indicator, once a gigaohm seal was obtained until at least 25 min after membrane breakthrough for whole-cell recordings. Each image was 512 × 512 pixels with a 1 μs pixel dwell time. In some cases the Alexa laser was used to also capture a transmission image to indicate the electrode and cell position ( Fig. 4a ). Pharmacological compounds Glutamate antagonists, D-(-)-2-Amino-5-phosphonopentanoic acid (D-APV; 10 μM) and 6-Cyano-7-nitroquinoxaline-2,3-dione (CNQX; 5 μM), the glycine antagonist, strychnine (0.3 μM) and the GABA A receptor antagonist bicuculline (10 μM) were purchased from Tocris Bioscience (Ellisville, MO, USA). TTX (1 μM) was purchased from Alomone Labs (Jerusalem, Israel). Stock solutions of these antagonists were prepared in water and were stored at −20 °C and working solutions were diluted with aCSF shortly before application to the bath. The antioxidant, NAC (1 mM) (Sigma) was prepared as a stock solution in water and dissolved in patch electrode solution on the day of the experiment. Mitochondrial poisons (antimycin-A, myxothiazol and rotenone) were purchased from Sigma, dissolved in dimethyl sulfoxide (DMSO) and diluted in water to workable stock concentrations and stored at −20 °C. The final maximum DMSO concentration (0.1% v/v) had no effect on mIPSCs. Although we tested antimycin-A at a range of concentrations (0.5–10 μM), we used a final concentration of 2 μM since it had a relatively fast onset time and was not detrimental to the cell’s health (based on the cell’s appearance and biophysical properties (i.e., input resistance, holding current)). In support of this, a comparable concentration of antimycin-A (1 μM) has been used in a similar electrophysiological study of ROS effects on nAChRs [42] . Mg-ATP was included in our patch electrode solution to avoid compromising Na + /K + ATPase function. For the Fenton reaction, H 2 O 2 (10 mM) was added to a solution of ascorbate (44 mM) and FeCl 3 ·6H 2 O (1 mM) at a 1:20 (v/v) dilution. This solution was added to the recording electrode solution at a 1:10 (v/v) dilution. The Fenton solution was prepared every 30 min from powdered ingredients at room temperature. Immunohistochemistry Three-week-old wild-type and α1-KO littermates were anesthetized with pentobarbital (50 mg kg −1 ) and perfusion-fixed with 4% paraformaldehyde solution in 0.1 M sodium phosphate buffer, pH 7.4. The brain was postfixed for 6 h, cryoprotected in 30% sucrose in phosphate-buffered saline, and cut parasagittally with a freezing microtome. Sections were pretreated with pepsin (0.15 mg ml −1 in 0.2 M HCl) for 10 min at 37 °C [43] to unmask synaptic proteins and incubated overnight in a mixture of antibodies against the α1 subunit (rabbit; custom-made), α3 subunit (guinea pig; custom-made) and gephyrin (mouse; mAb7a, Synaptic Systems, Göttingen, Germany), followed by three washes and incubation in secondary antibodies coupled to Alexa488, Cy3 and Cy5 (Jackson Immunoresearch, West Grove, PA, USA). Images were acquired by confocal laser scanning microscopy (Zeiss LSM700, Carl Zeiss MicroImaging GmbH, Germany) using a × 40 objective (N.A. 1.4). Stacks of 3–10 confocal images spaced by 0.5 μm were projected for display. How to cite this article : Accardi, M. V. et al. Mitochondrial reactive oxygen species regulate the strength of inhibitory GABA-mediated synaptic transmission. Nat. Commun. 5:3168 doi: 10.1038/ncomms4168 (2014).